Rapid14C excursion at 3372-3371 BCE not observed at two different locations 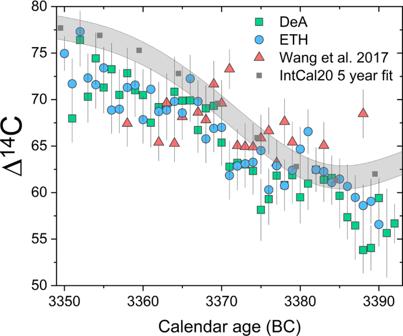Fig. 1: Measurements of Δ14C (in ‰) vs. dendrochronologically derived calendar age for samples of bristlecone pine (measured in Debrecen, DeA) and European Oak (measured in Zürich, ETH), compared to the reported Δ14C results for Chinese wingnut of Wang et al.8. In the case of the wingnut samples, the age reported by ref.8is used as the age on the ordinate axis. The green squares show data from Debrecen, the blue circles data from ETH, and the red triangles show the results of Wang et al.8. The gray area shows the international calibration curve (IntCal20)11with 1σerror, which is based on a spline fit to the IntCal20 at 5-year resolution. 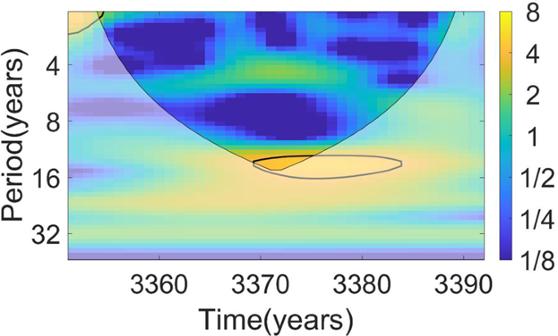Fig. 2: Wavelet analysis of the bristlecone pine14C series. Shades denote the dimensionless continuous wavelet transform power-spectrum density. The color bar placed on the right represents the squared power of the wavelet transform and the numbers indicate the spectrum power level (dimensionless). High values in a few time intervals (x-axis) with some periodicity (y-axis) show that the amplitude of a signal with that periodicity emerges from noise in those years. The black contour denotes the 5% significance level against red noise. The area where edge effect influence distorts the picture is shown in lighter shades. The signal attributable to solar the solar cycle is marked with yellow fields. The black line outlines the variance significant relative to red noise. A similar result can be obtained for the European Oak series (shown in Supplementary Fig.1). The bristlecone wood specimen used in this study (Supplementary Fig. 2 ) was collected by M. Salzer in July 2003 at the elevation of 3575 m asl on the Sheep Mountain ridge (37.53475N and 118.20045W). The ring widths of this specimen were measured on a Lintab system. The 328-year ring series is correlated with the 6422-year master chronology from Sheep Mountain spanning from 4408 BCE to 2014 CE, which is composed of tree rings from remnant wood and overlaps with rings from living trees [16] . The Sheep Mountain chronology also correlates well with two other long bristlecone tree-ring chronologies from the same mountain range confirming the dating accuracy of the chronology. Dating SH146-2003 was assigned using correlation of ring widths between 50-year segments and the master SHP mountain chronology lagged successively by 25 years with statistical verification using COFECHA12K version 6.06P, which uses multiple parametric statistics to examine the quality of various fits [20] . Second checks on dating were confirmed through the presence/absence of sub-annual ring features, such as frost rings. Further details of master chronology construction are published in refs. [16] , [20] . The cross-dating and the master chronology development were performed at the Laboratory of Tree-Ring Research, University of Arizona. The SH146-2003 remnant specimen has no locally absent rings and includes a very prominent frost ring formed in 3458 BCE that is also present in the same year in one other sample of the master chronology. The annual growth layers were separated through cutting with a razor blade and grounded to 20-μm mesh. Each powdered sample was converted to α-cellulose using standard procedures [23] , [24] . The oak sample (CHEY1-17) originated from an accumulation of 17 subfossil oak trunks found during gravel extraction in the Moselle River valley (48.9405N, 6.0586E) in 2011 (Supplementary Fig. 3 ). Tree-ring widths were measured to an accuracy of 1/100 mm using a stereo microscope and a measuring system. The annually resolved tree-ring width series of 14 tree trunks are synchronized into a 247-year mean chronology. This site chronology is overlapped with the master oak chronology for South Germany [17] . After 10-year smoothing spline transformation, these two chronologies correlate at R = 0.53 for the common period from 3405 BCE to 3159 BCE. The cross-dating was performed at University of Freiburg. Bristlecone cellulose samples were combusted to CO 2 and converted to graphite, and 14 C dating was performed using the 200 kV MICADAS (Mini Carbon Dating System, Ion Plus AG, Dietikon, Switzerland) at the Institute for Nuclear Research in Debrecen, Hungary [23] . Sample calculation and data reduction were done using the standard BATS software [25] . Oak samples were converted to α-cellulose using the procedures described in ref. [24] , and the accelerator mass spectrometer (AMS) samples were converted to graphite using the automated graphitization equipment (AGE-3) system at the Swiss Federal Institute of Technology, Zürich. Samples were measured on a MICADAS 200 kV AMS of the same design and software [25] as the Debrecen machine.